Arabidopsisnitrate reductase activity is stimulated by the E3 SUMO ligase AtSIZ1 Small ubiquitin-related modifier (SUMO) is a small polypeptide that modulates protein activity and regulates hormone signalling, abiotic and biotic responses in plants. Here we show that AtSIZ regulates nitrogen assimilation in Arabidopsis through its E3 SUMO ligase function. Dwarf plants of siz1-2 flower early, show abnormal seed development and have high salicylic acid content and enhanced resistance to bacterial pathogens. These mutant phenotypes are reverted to wild-type phenotypes by exogenous ammonium but not by nitrate, phosphate or potassium. Decreased nitrate reductase activity in siz1-2 plants resulted in low nitrogen concentrations, low nitric oxide production and high nitrate content in comparison with wild-type plants. The nitrate reductases, NIA1 and NIA2, are sumoylated by AtSIZ1, which dramatically increases their activity. Both sumoylated and non-sumoylated NIA1 and NIA2 can form dimers. Our results indicate that AtSIZ1 positively controls nitrogen assimilation by promoting sumoylation of NRs in Arabidopsis . Nitrogen is one of the most important inorganic nutrients and a major component of nucleic acids, proteins, various cofactors and secondary metabolites. Plants have evolved to utilize nitrate as a source of environmental nitrogen, and nitrate serves as a potent signal that regulates nitrogen and carbon metabolism as well as organ growth and development [1] , [2] , [3] , [4] . Nitrate from the soil is transported actively into cells by a nitrate transporter and is reduced sequentially to ammonia, which enters the amino-acid pool primarily via the action of glutamine synthetase. Homodimers of plant nitrate reductase (NR) catalyse the NAD(P)H-dependent reduction of nitrate to nitrite [5] , [6] , which is reduced further to ammonium by NR in the second step of the nitrate assimilation pathway [7] . The Arabidopsis genome contains two NR genes, NIA1 and NIA2 . The nia1/nia2 double mutant flowers early [8] . Small ubiquitin-related modifier (SUMO), a key regulator of biological processes, is covalently conjugated to a lysine residue in a substrate protein via a reversible posttranslational modification process that is facilitated by E3 SUMO ligases [9] . As in other eukaryotes, SUMO modification in plants has been implicated in numerous basic cellular processes, such as stress and defence responses and the regulation of flowering [10] , [11] , [12] , [13] , [14] , [15] , [16] , [17] , [18] . AtSIZ1 is an SP-RING-finger protein that contains a SAP domain and a zinc-finger Miz domain. AtSIZ1 is a key regulator of signalling pathways that mediate responses to nutrient deficiency and environmental stresses [14] , [15] , [16] , [17] , [19] , [20] , [21] , [22] . The observation that mutations in AtSIZ1 result in dwarf plants with smaller leaves indicates that AtSIZ1 also has a role in vegetative growth and development [16] , [17] , [23] . Despite the involvement of sumoylation in a wide range of physiological processes, only a few Arabidopsis proteins, including the SUMO machinery proteins AtSIZ1 and AtSCE1, have been experimentally demonstrated to be sumoylated [24] . Very recently, two groups have identified massive SUMO conjugates by proteomics methods [25] and yeast two-hybrid screening [26] in Arabidopsis under non-stress and stress conditions. The results indicated that sumoylation can regulate diverse biological processes, although the functional consequences of this modification were not fully characterized. Nitrogen assimilation is a fundamental biological process that has a marked effect on plant productivity, biomass and crop yield. NR is a key enzyme in a plant's nitrogen assimilation pathway. However, few components that influence NR activity have been identified [27] , [28] , and NR regulation at the posttranslational level has not been well characterized. Here, we investigated the contribution of AtSIZ1-mediated nitrate reduction to nitrogen assimilation in Arabidopsis . siz1 mutants were recovered as to the wild-type (WT) phenotype when supplemented with exogenous ammonium and NR activity of NIA1 and NIA2 was increased by sumoylation through E3 ligase activity of AtSIZ1. Our results provide the first biochemical evidence that sumoylation is a critical protein modification required for the regulation of NR activity. Ammonium recovers the siz1-2 mutant phenotype The Arabidopsis siz1-2 mutants display a dwarf phenotype, early flowering and abnormal seed development. We examined the capacity of Arabidopsis siz1-2 mutants to recover growth and normal development in response to the provision of a nitrogen source and/or supplementation with phosphate or potassium, as these factors are essential for plant growth and development. During vegetative growth, the WT phenotype was restored with the use of ammonium, but not nitrate, as a nitrogen source ( Fig. 1 ; Supplementary Fig. S1 ). During the reproductive phase, siz1-2 mutant phenotypes such as short silique length, lower seed number (about 50% of WT) and sterility were restored to WT phenotypes with ammonium ( Supplementary Fig. S2 and Table S1 ). This result indicates that the mutant reproductive phenotypes are caused by impairment of the nitrate reduction pathway because of the AtSIZ1 mutation. 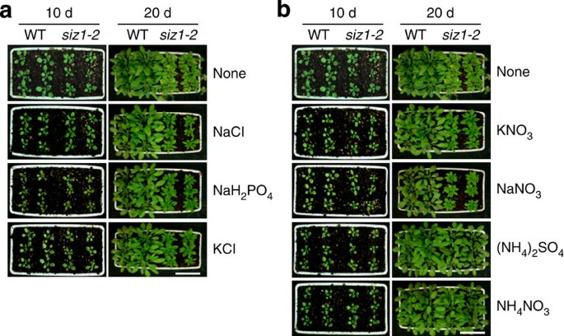Figure 1: Growth patterns of WT andsiz1-2plants and the effect of nitrogen sources on their growth. (a) After germination on MS media, seedlings were transferred to soil and treated with 5 mM phosphate and potassium. (b)Seedlings were also treated with 5 mM of each nitrogen source for 10 and 20 days. The growth ofsiz1-2plants was recovered by ammonium sources such as (NH4)2SO4and NH4NO3, but not by nitrate sources (such as KNO3or NaNO3), phosphate or potassium. Scale bar, 5 cm. Figure 1: Growth patterns of WT and siz1-2 plants and the effect of nitrogen sources on their growth. ( a ) After germination on MS media, seedlings were transferred to soil and treated with 5 mM phosphate and potassium. ( b) Seedlings were also treated with 5 mM of each nitrogen source for 10 and 20 days. The growth of siz1-2 plants was recovered by ammonium sources such as (NH 4 ) 2 SO 4 and NH 4 NO 3 , but not by nitrate sources (such as KNO 3 or NaNO 3 ), phosphate or potassium. Scale bar, 5 cm. Full size image NR is the only enzyme to catalyse the conversion of nitrite to nitric oxide (NO) in several higher plants [29] , [30] , [31] , [32] , although the primary function of NR is nitrogen assimilation through the reduction of nitrate to nitrite. Low levels of NO in the NR double mutant nia1/nia2 have been reported to cause early flowering [8] , [33] , similar to siz1-2 plants [21] . Interestingly, ammonium-treated siz1-2 plants showed restored flowering time ( Supplementary Fig. S1 ), implying that nitrate reduction is impaired in siz1-2 . Decreased nitrogen content and NR activity in siz1-2 plants We assessed NR activity in siz1-2 plants using chlorate, the chlorine analogue of nitrate, which is reduced to the toxic chlorite by NR. Phenotypic analysis revealed a less severe inhibition of growth of chlorate-treated siz1-2 plants compared with WT plants ( Supplementary Fig. S3 ). This result indicates that the siz1-2 plants have low NR activity. Further analysis showed that NR activity was decreased in both the leaves and roots of the siz1-2 plants compared with WT plants ( Fig. 2a,b ). 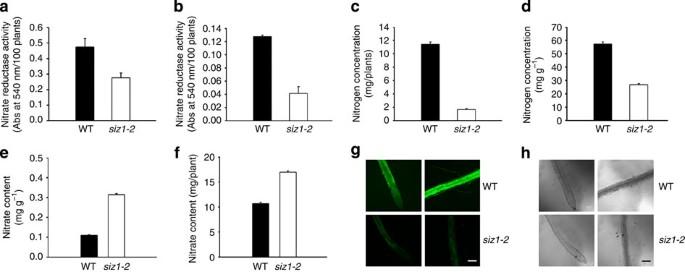Figure 2: NR activity is decreased insiz1-2plants. Nitrogen and nitrate concentrations and NR activity were measured in the leaves of WT andsiz1-2plants. NR activities in the leaves (a) or roots (b) of 100 WT orsiz1-2plants. Nitrogen amounts per plant (c) or per gram (d) of WT andsiz1-2plants. Nitrate amount calculated per gram (e) or per plant (f). Results ina–fare shown as means±s.d. ofn=3 (a,b,e,f) orn=5 (c,d).In situNO was measured in the roots of WT andsiz1-2plants, which were labelled with DAF-2DA and visualized with fluorescent (g) or light (h) microscopy. Scale bar, 100 μm. Figure 2: NR activity is decreased in siz1-2 plants. Nitrogen and nitrate concentrations and NR activity were measured in the leaves of WT and siz1-2 plants. NR activities in the leaves ( a ) or roots ( b ) of 100 WT or siz1-2 plants. Nitrogen amounts per plant ( c ) or per gram ( d ) of WT and siz1-2 plants. Nitrate amount calculated per gram ( e ) or per plant ( f ). Results in a – f are shown as means±s.d. of n =3 ( a , b , e , f ) or n =5 ( c , d ). In situ NO was measured in the roots of WT and siz1-2 plants, which were labelled with DAF-2DA and visualized with fluorescent ( g ) or light ( h ) microscopy. Scale bar, 100 μm. Full size image On the basis of the low NR activity of siz1-2 plants, nitrate reduction and nitrogen assimilation were assessed by measuring the nitrogen and nitrate concentrations and NO production in the mutant plants. As expected, nitrogen content was low ( Fig. 2c,d ; Supplementary Table S2 ) and nitrate content was high in siz1-2 plants ( Fig. 2e,f ). In addition, NO production was decreased in siz1-2 plants ( Fig. 2g,h ), which supports the previous finding that NO accumulation is mediated by an NR-associated pathway [34] . E3 SUMO ligase activity of AtSIZ1 on NIA1 and NIA2 Our results imply that AtSIZ1 may modulate the activity or stability of NIA1 and NIA2 by acting as an E3 SUMO ligase. The deduced amino-acid sequences of the NRs, NIA1 and NIA2, revealed that both proteins have putative sumoylation sites (ψKXE), which were located at lysine 356 (K356) of NIA1 and lysine 353 (K353) of NIA2 ( Supplementary Fig. S4 ). Therefore, to evaluate the possible interaction between AtSIZ1 and NIA1 or NIA2, glutathione sulphur transferase (GST)-tagged AtSIZ1 and histidine-tagged NIA1 or NIA2 were overexpressed in Escherichia coli and purified with glutathione and Ni 2+ -NTA resins, respectively. In vitro pull-down of His 6 -NIA1 or His 6 -NIA2 with GST and GST-AtSIZ1 revealed that AtSIZ1 interacts with both His 6 -NIA1 and His 6 -NIA2, whereas the resin or GST alone did not interact with either His 6 -NIA1 or His 6 -NIA2 ( Supplementary Fig. S5a ). These specific interactions were also examined by yeast two-hybrid assays with AtSIZ1 and NIA1 or NIA2 . These genes were cloned into a yeast expression vector containing either an activation domain or a binding domain. A strong interaction between AtSIZ1 and NIA1 or NIA2 was detected ( Supplementary Fig. S5b ), similar to the results of the pull-down experiment. On the basis of the interaction between AtSIZ1 and NIA1 or NIA2, we examined the possibility that the NRs could be substrates for AtSIZ1. His 6 -AtSAE1b, His 6 -AtSAE2, His 6 -AtSCE1, His 6 -AtSUMO1, GST-AtSIZ1, GST-NIA1-Myc and GST-NIA2-Myc were overexpressed in E. coli and purified with Ni 2+ -NTA or glutathione resins ( Fig. 3a ). Then, the recombinant proteins were applied to the in vitro sumoylation reactions. Both NIA1 and NIA2 were sumoylated by AtSIZ1 in a reaction that was dependent on E1 and E2 activities ( Fig. 3b ). 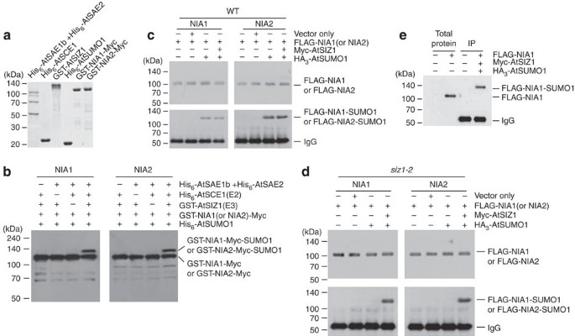Figure 3: NIA1 and NIA2 are sumoylated by AtSIZ1. (a) PurifiedArabidopsisHis-AtSAE1b, His-AtSAE2, His6-AtSCE1, GST-AtSIZ1, His6-AtSUMO1 and GST-NIA1 (or NIA2)-Myc were separated by 11% SDS–PAGE. (b)Sumoylation of GST-NIA1 (or NIA2)-Myc was assayed in the presence or absence of His6-AtSAE1b, His6-AtSAE2, His6-AtSCE1, His6-AtSUMO1 and GST-AtSIZ1. After the reaction, sumoylated NIA1 or NIA2 was detected by immunoblotting with an anti-Myc antibody. AtSIZ1-mediated E3 sumoylation of NIA1 or NIA2 was examined inArabidopsis. Leaves of WT (c) orsiz1-2plants (d) were infiltrated with35S-Myc-AtSIZ1,35S-HA3-AtSUMO1and35S-FLAG-NIA1(orNIA2), as indicated. After incubation for 3 days, FLAG-NIA1 (or NIA2) was detected by immunoblotting with an anti-FLAG antibody. Sumoylated NIA1 or NIA2 was detected by immunoblotting with an anti-FLAG antibody after IP with an anti-HA antibody. (e) To confirm the size of the non-sumoylated or sumoylated form of NIA1, total proteins were extracted from the leaves of WT plants infiltrated without or with35S-FLAG-NIA1construct. Total proteins were also extracted from the leaves of WT plants infiltrated without or with35S-Myc-AtSIZ1,35S-HA3-AtSUMO1and35S-FLAG-NIA1, and were immunoprecipitated with an anti-HA antibody. Total proteins or immunoprecipitated proteins were separated by 11% SDS–PAGE and detected by immunoblotting using an anti-FLAG antibody. IgG, immunoglobulin G. Figure 3: NIA1 and NIA2 are sumoylated by AtSIZ1. ( a ) Purified Arabidopsis His-AtSAE1b, His-AtSAE2, His 6 -AtSCE1, GST-AtSIZ1, His 6 -AtSUMO1 and GST-NIA1 (or NIA2)-Myc were separated by 11% SDS–PAGE. ( b) Sumoylation of GST-NIA1 (or NIA2)-Myc was assayed in the presence or absence of His 6 -AtSAE1b, His 6 -AtSAE2, His 6 -AtSCE1, His 6 -AtSUMO1 and GST-AtSIZ1. After the reaction, sumoylated NIA1 or NIA2 was detected by immunoblotting with an anti-Myc antibody. AtSIZ1-mediated E3 sumoylation of NIA1 or NIA2 was examined in Arabidopsis . Leaves of WT ( c ) or siz1-2 plants ( d ) were infiltrated with 35S-Myc-AtSIZ1 , 35S-HA 3 -AtSUMO1 and 35S-FLAG-NIA1 (or NIA2 ), as indicated. After incubation for 3 days, FLAG-NIA1 (or NIA2) was detected by immunoblotting with an anti-FLAG antibody. Sumoylated NIA1 or NIA2 was detected by immunoblotting with an anti-FLAG antibody after IP with an anti-HA antibody. ( e ) To confirm the size of the non-sumoylated or sumoylated form of NIA1, total proteins were extracted from the leaves of WT plants infiltrated without or with 35S-FLAG-NIA1 construct. Total proteins were also extracted from the leaves of WT plants infiltrated without or with 35S-Myc-AtSIZ1 , 35S-HA 3 -AtSUMO1 and 35S-FLAG-NIA1 , and were immunoprecipitated with an anti-HA antibody. Total proteins or immunoprecipitated proteins were separated by 11% SDS–PAGE and detected by immunoblotting using an anti-FLAG antibody. IgG, immunoglobulin G. Full size image To test whether AtSIZ1 functions as an E3 SUMO ligase for NIA1 and NIA2 in plants, 35S-HA 3 -SUMO1 , 35S-Myc-AtSIZ1 and 35S-FLAG-NIA1 or 35S-FLAG-NIA2 constructs were coinfiltrated into the leaves of WT or siz1-2 plants. The sumoylation of NIA1 or NIA2 was examined by immunoblotting against an anti-FLAG antibody after immunoprecipitation (IP) with an anti-HA antibody. Notably, sumoylated NIA1 and NIA2 were detected clearly in both WT and siz1-2 plants when infiltrated with 35S-Myc-AtSIZ1 ( Fig. 3c ), while they were not detected in siz1-2 plants that were not infiltrated with 35S-Myc-AtSIZ1 ( Fig. 3d ). This result indicates that AtSIZ1 functions as an E3 SUMO ligase for NIA1 and NIA2. The size of the non-sumoylated or sumoylated form of NIA1 was also compared to confirm whether it is a real sumoylated form. Only NIA1 was checked, because both NIA1 and NIA2 have the same sumoylation patterns and similar molecular weight ( Fig. 3b–d ). Migration of the sumoylated form was retarded about 20 kDa on SDS–polyacrylamide gel ( Fig. 3e ), which is a typical feature of sumoylated protein. This system was also applied to Nicotiana benthamiana to confirm the sumoylation results, and the results showed that both NIA1 and NIA2 were sumoylated ( Supplementary Fig. S6 ), as in the Arabidopsis system. To identify the sumoylation sites in NIA1 and NIA2, mutant derivatives (mNIA1 and mNIA2) with K356R and K353R mutations in NIA1 and NIA2, respectively, were generated ( Supplementary Fig. S7a ). These mutations blocked AtSIZ1-mediated sumoylation in vitro ( Supplementary Fig. S7b ). These in vitro results were confirmed in vivo by transient expression in the leaves of WT and siz1-2 plants coinfiltrated with the 35S-FLAG-NIA1 (or mNIA1) and 35S-FLAG-NIA2 (or mNIA2 ) constructs, as above. The results obtained with coinfiltrated plants were consistent with the in vitro data ( Supplementary Fig. S8a,b ). K-to-R substitutions in the sumoylation motifs effectively blocked the formation of isopeptide linkages between SUMO and the target proteins [35] . Our combined results indicate that K356 and K353 are the principal sites of SUMO conjugation in NIA1 and NIA2, respectively. Increase of NR activities by sumoylation Most of the proteins that are posttranslationally modified by small or large molecules are functionally regulated. We investigated the effect of the sumoylation of NIA1 and NIA2 on their NR activities. Because the NRs function as dimers, the effect of sumoylation on the dimerization of NIA1 or NIA2 was examined. To examine whether non-sumoylated NIA1 or NIA2 forms dimers, IP was performed using the leaf extracts of Arabidopsis coinfiltrated with various combinations of 35S-HA 3 -AtSUMO1 , 35S-FLAG-NIA1 (or mNIA1) and 35S-Myc-NIA1 (or mNIA1) , or 35S-FLAG-NIA2 (or mNIA2) and 35S-Myc-NIA2 (or mNIA2) . The results revealed that non-sumoylated NIA1 or NIA2 can form homodimers ( Supplementary Fig. S9 ). To examine whether sumoylated NIA1 or NIA2 forms dimers, IP was performed using the leaf extracts of N. benthamiana coinfiltrated with various combinations of XVE-His 6 -HA 3 -AtSUMO1/35S-FLAG-NIA1 (or mNIA1 ) or XVE-His 6 -HA 3 -AtSUMO1/35S-Myc-NIA1 (or mNIA1 ) and XVE-His 6 -HA 3 -AtSUMO1/35S-FLAG-NIA2 (or mNIA2 ) or XVE-His 6 -HA 3 -AtSUMO1/35S-Myc-NIA2 (or mNIA2 ). After overnight incubation, the leaves were injected again with 10 μM β-estradiol, because AtSUMO1 expression is induced by β-estradiol. The results indicated that sumoylated NIA1 or NIA2 can form homodimers ( Supplementary Fig. S10a-d ). Next, the effect of sumoylation on the NR activities of NIA1 and NIA2 was assessed by measuring the amount of nitrite produced from nitrate after the in vitro sumoylation reactions ( Fig. 4a ). After 2 h, the nitrite concentration was increased significantly in the reaction mix containing sumoylated NIA1 or NIA2, but was increased slightly in the reaction mix containing non-sumoylated proteins, compared with reaction mix without NIA1 or NIA2 ( Fig. 4b ). These results indicate that SUMO conjugation activates the NR activities of NIA1 or NIA2. 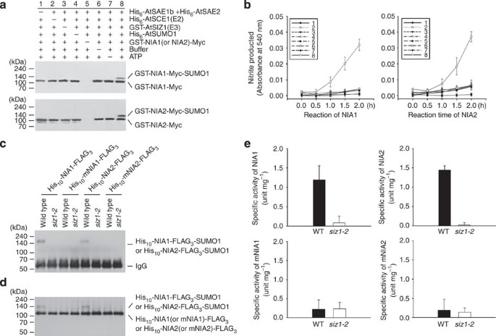Figure 4: Effect of SUMO conjugation on NR activity. The NR activity was assayed as a function of nitrite production. (a) Sumoylation of NIA1 or NIA2in vitro. Afterin vitrosumoylation reactions, nitrate was added into the reaction mixtures and further incubated for the indicated times. Products were separated on SDS–PAGE and transferred onto a nitrocellulose membrane. Sumoylation of NIA1 or NIA2 was examined by immunoblotting using an anti-Myc antibody. (b) The effect of sumoylation on NR activity was examined in either NIA1 or NIA2. Bar numbers indicate the reaction numbers shown ina. Nitrite concentration was measured at 540 nm. (c,d) Sumoylation of NIA1 or NIA2in vivo. Leaves of WT orsiz1-2plants were infiltrated with35S-HA3-AtSUMO1and35S-His10-NIA1(ormNIA1)-FLAG3or35S-His10-NIA2(ormNIA2)-FLAG3, as indicated. After incubation for 3 days, the infiltrated leaves were collected. Sumoylated His10-NIA1 (or NIA2)-FLAG3-SUMO1 was detected with an anti-FLAG antibody after IP with an anti-HA antibody (c). Total proteins were extracted. Histidine-tagged proteins were purified with a Ni2+-NTA column, followed by quantification of protein concentration with the Bradford method. His10-NIA1 (or mNIA1)-FLAG3or His10-NIA2 (or mNIA2)-FLAG3and/or sumoylated His10-NIA1 (or NIA2)-FLAG3-SUMO1 were detected by immunoblotting with an anti-FLAG antibody (d). IgG, immunoglobulin G. (e) Effect of sumoylation on NR activityin vivo. Specific activities of NIA1 and NIA2 were measured with the column-purified NIA1 or NIA2 from WT orsiz1-2plants shown ind. Results are expressed as means±s.d. (n=3). Figure 4: Effect of SUMO conjugation on NR activity. The NR activity was assayed as a function of nitrite production. ( a ) Sumoylation of NIA1 or NIA2 in vitro . After in vitro sumoylation reactions, nitrate was added into the reaction mixtures and further incubated for the indicated times. Products were separated on SDS–PAGE and transferred onto a nitrocellulose membrane. Sumoylation of NIA1 or NIA2 was examined by immunoblotting using an anti-Myc antibody. ( b ) The effect of sumoylation on NR activity was examined in either NIA1 or NIA2. Bar numbers indicate the reaction numbers shown in a . Nitrite concentration was measured at 540 nm. ( c , d ) Sumoylation of NIA1 or NIA2 in vivo . Leaves of WT or siz1-2 plants were infiltrated with 35S-HA 3 -AtSUMO1 and 35S-His 10 -NIA1 (or mNIA1)-FLAG 3 or 35S-His 10 -NIA2 (or mNIA2)-FLAG 3 , as indicated. After incubation for 3 days, the infiltrated leaves were collected. Sumoylated His 10 -NIA1 (or NIA2)-FLAG 3 -SUMO1 was detected with an anti-FLAG antibody after IP with an anti-HA antibody ( c ). Total proteins were extracted. Histidine-tagged proteins were purified with a Ni 2+ -NTA column, followed by quantification of protein concentration with the Bradford method. His 10 -NIA1 (or mNIA1)-FLAG 3 or His 10 -NIA2 (or mNIA2)-FLAG 3 and/or sumoylated His 10 -NIA1 (or NIA2)-FLAG 3 -SUMO1 were detected by immunoblotting with an anti-FLAG antibody ( d ). IgG, immunoglobulin G. ( e ) Effect of sumoylation on NR activity in vivo . Specific activities of NIA1 and NIA2 were measured with the column-purified NIA1 or NIA2 from WT or siz1-2 plants shown in d . Results are expressed as means±s.d. ( n =3). Full size image The effect of sumoylation on the specific activities of NIA1 and NIA2 was further examined using the leaves of WT or siz1-2 plants coinfiltrated with various combinations of 35S-HA 3 -AtSUMO1 and 35S-His 10 -NIA1 (or mNIA1)-FLAG 3 or 35S-His 10 -NIA2 (or mNIA2)-FLAG 3 . Sumoylated NIA1 and NIA2 bands were seen after IP ( Fig. 4c ). The specific activity of sumoylated or non-sumoylated NIA1 and NIA2 purified with nickel resins was measured ( Fig. 4d ). The specific activities were much higher in WT plants expressing sumoylated NIA1 or NIA2 than in siz1-2 plants expressing only non-sumoylated NIA1 or NIA2 ( Fig. 4e ). However, the values were very low and similar in both WT and siz1-2 plants expressing only mNIA1 or mNIA2, which shows that the NIA1 and NIA2 activities are increased significantly by AtSIZ1-mediated sumoylation. Increased stability of NRs by AtSIZ1 SUMO conjugation is known to stabilize target proteins in several systems. To investigate whether the stabilities of NIA1 and NIA2 are regulated by AtSIZ1 activity, NIA1 and NIA2 protein levels in WT, siz1-2 , nia1 , nia2 and nia1 / nia2 plants were assessed by immunoblotting with an antibody to cucumber NR, which crossreacts with both NIA1 and NIA2. The reductase levels were about twofold higher in WT and siz1-2 plants than in nia1 or nia2 plants ( Fig. 5a,b ). 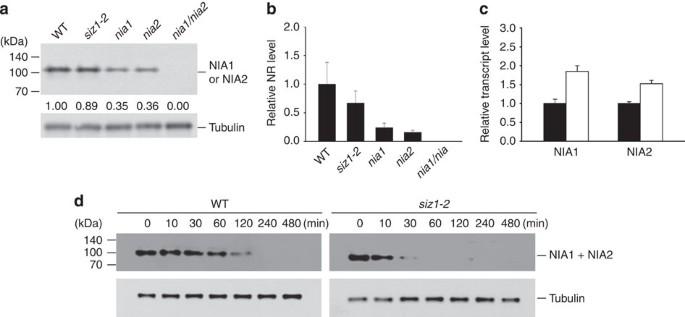Figure 5: Effect of AtSIZ1 on NR levels. (a,b) Total proteins were extracted from the leaves of WT,siz1-2,nia1,nia2andnia1/nia2plants. The NIA1 or NIA2 proteins were detected by immunoblotting with a cucumber anti-NR antibody. Tubulin levels were used as loading controls. Experiments were carried out four times, and one of the immunoblotting results is shown (a). Numbers under lanes indicate relative intensities. Mean values of the intensities were calculated and used to draw the graph (b). Results are shown as means±s.e. (n=4). (c) Total RNA was isolated from cycloheximide-treated WT andsiz1-2plants. Transcript levels of NIA1 and NIA2 were examined by real-time RT–PCR with gene-specific primers. Black and white bars indicate WT andsiz1-2, respectively. (d) Total proteins were extracted from cycloheximide-treated WT andsiz1-2plants for the indicated time. The NRs were detected by immunoblotting with the cucumber anti-NR antibody. Tubulin levels were used as loading controls. Figure 5: Effect of AtSIZ1 on NR levels. ( a , b ) Total proteins were extracted from the leaves of WT, siz1-2 , nia1 , nia2 and nia1 / nia2 plants. The NIA1 or NIA2 proteins were detected by immunoblotting with a cucumber anti-NR antibody. Tubulin levels were used as loading controls. Experiments were carried out four times, and one of the immunoblotting results is shown ( a ). Numbers under lanes indicate relative intensities. Mean values of the intensities were calculated and used to draw the graph ( b ). Results are shown as means±s.e. ( n =4). ( c ) Total RNA was isolated from cycloheximide-treated WT and siz1-2 plants. Transcript levels of NIA1 and NIA2 were examined by real-time RT–PCR with gene-specific primers. Black and white bars indicate WT and siz1-2 , respectively. ( d ) Total proteins were extracted from cycloheximide-treated WT and siz1-2 plants for the indicated time. The NRs were detected by immunoblotting with the cucumber anti-NR antibody. Tubulin levels were used as loading controls. Full size image NIA1 and NIA2 transcript levels were examined by real-time reverse transcription (RT)–PCR using WT and siz1-2 plants treated with cycloheximide. Their transcript levels were much higher in the siz1-2 mutant than in WT plants ( Fig. 5c ), although their protein levels were very similar in the WT and siz1-2 plants ( Fig. 5a,b ). This finding indicates that the stability of the NIA1 and NIA2 proteins can be affected by AtSIZ1. Next, the decays of NIA1 and NIA2 were evaluated in the presence of cycloheximide to compare the degradation rates between WT and siz1-2 plants. The degradations of NIA1 and NIA2 were much faster in siz1-2 than in WT plants ( Fig. 5d ), which indicates that NRs must be stabilized by AtSIZ1. The AtSIZ1 transcript and protein levels did not change significantly with nitrate or ammonium treatment ( Fig. 6a–d ). This result indicates that the amount and stability of AtSIZ1 were unaffected by these treatments. 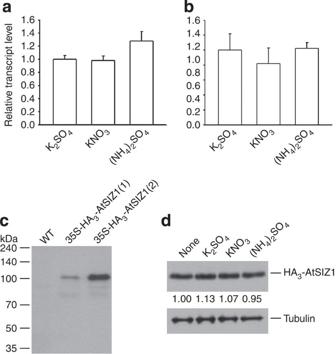Figure 6: Effect of nitrate or ammonium ion onAtSIZ1transcript and AtSIZ1 protein levels. (a,b) Effect of nitrate or ammonium ion on theAtSIZ1transcript level. The leaves (a) and roots (b) of WT plants were treated with 5 mM KNO3or (NH4)2SO4, and the transcript level ofAtSIZ1was examined by real-time RT–PCR. Results are expressed as means±s.e. (n=3). (c) Transgenic plants overexpressingHA3-AtSIZ1. Total proteins were extracted from transgenic plants harbouring35S-HA3-AtSIZ1, and the HA3-AtSIZ1 protein was detected by immunoblotting with an anti-HA antibody. Numbers within parentheses indicate independent transgenic lines. Transgenic line (number 2) with high HA3-AtSIZ1 protein was chosen for further experimentation. (d) Effect of nitrate or ammonium sources on AtSIZ1 stability transgenic plants were treated with 5 mM KNO3or (NH4)2SO4. The HA3-AtSIZ1 protein levels were detected by immunoblotting with an anti-HA antibody. Tubulin levels were used as loading controls. Numbers under lanes indicate relative intensities. Figure 6: Effect of nitrate or ammonium ion on AtSIZ1 transcript and AtSIZ1 protein levels. ( a , b ) Effect of nitrate or ammonium ion on the AtSIZ1 transcript level. The leaves ( a ) and roots ( b ) of WT plants were treated with 5 mM KNO 3 or (NH 4 ) 2 SO 4 , and the transcript level of AtSIZ1 was examined by real-time RT–PCR. Results are expressed as means±s.e. ( n =3). ( c ) Transgenic plants overexpressing HA 3 -AtSIZ1 . Total proteins were extracted from transgenic plants harbouring 35S-HA 3 -AtSIZ1 , and the HA 3 -AtSIZ1 protein was detected by immunoblotting with an anti-HA antibody. Numbers within parentheses indicate independent transgenic lines. Transgenic line (number 2) with high HA 3 -AtSIZ1 protein was chosen for further experimentation. ( d ) Effect of nitrate or ammonium sources on AtSIZ1 stability transgenic plants were treated with 5 mM KNO 3 or (NH 4 ) 2 SO 4 . The HA 3 -AtSIZ1 protein levels were detected by immunoblotting with an anti-HA antibody. Tubulin levels were used as loading controls. Numbers under lanes indicate relative intensities. Full size image Expression of nitrate assimilation genes in siz1-2 mutants The above results indicate that AtSIZ1 has a role in plant development by regulating nitrate reduction through its E3 SUMO ligase activity. However, the developmental defect of siz1-2 plants also could be due to deficiencies in nitrate uptake, nitrate to nitrite reduction, or formation of glutamate or glutamine caused by the downregulation of nitrate metabolism-related genes. The expression levels of genes encoding the nitrate transporters NRT1.1 and NRT1.2 , the ammonium transporter AtAMT1 , the NRs NIA1 and NIA2 , and the glutamine and glutamate synthases GS and GOGAT were investigated in WT and siz1-2 plants. The relative transcript levels of these genes were higher in the leaves and roots of siz1-2 plants than in those of WT plants ( Fig. 7a–g ). This result indicates that the phenotype of the siz1-2 plants cannot be attributed to a repression of the genes tested. 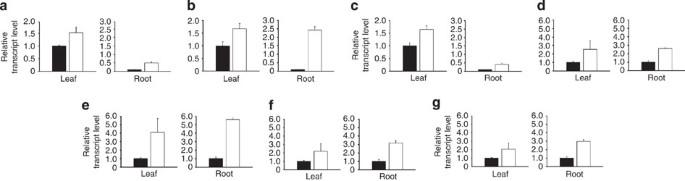Figure 7: Relative transcript levels of nitrate metabolism-related genes. Total RNAs were isolated from the leaves and roots of WT andsiz1-2plants. The mRNA levels were examined by real-time RT–PCR with gene-specific primers.NRT1-1(a), nitrate transporter 1-1;NRT1-2(b), nitrate transporter 1-2;AtAMT1(c),Arabidopsisammonium transporter 1;NIA1(d), nitrate reductase 1;NIA2(e), nitrate reductase 2;GS(f), glutamine synthase;GOGAT(g), glutamine oxoglutarate aminotransferase. Results are expressed as means±s.e. (n=3). Black and white bars indicate WT andsiz1-2, respectively. Figure 7: Relative transcript levels of nitrate metabolism-related genes. Total RNAs were isolated from the leaves and roots of WT and siz1-2 plants. The mRNA levels were examined by real-time RT–PCR with gene-specific primers. NRT1-1 ( a ), nitrate transporter 1-1; NRT1-2 ( b ), nitrate transporter 1-2; AtAMT1 ( c ), Arabidopsis ammonium transporter 1; NIA1 ( d ), nitrate reductase 1; NIA2 ( e ), nitrate reductase 2; GS ( f ), glutamine synthase; GOGAT ( g ), glutamine oxoglutarate aminotransferase. Results are expressed as means±s.e. ( n =3). Black and white bars indicate WT and siz1-2 , respectively. Full size image Recovery of disease resistance by ammonium in siz1-2 plants A recent study showed that the expression of the pathogenesis-related genes PR1 and PR2 was induced in siz1-2 plants by high salicylic acid (SA) levels [17] . Thus, PR1 and PR2 expression levels and free and glucosyl SA levels were examined in the leaves of WT and siz1-2 plants grown with KNO 3 or (NH 4 ) 2 SO 4 in soil. The transcript levels of PR1 and PR2 ( Fig. 8a,b ) and SA levels ( Fig. 8c,d ) were recovered to WT levels under these conditions. 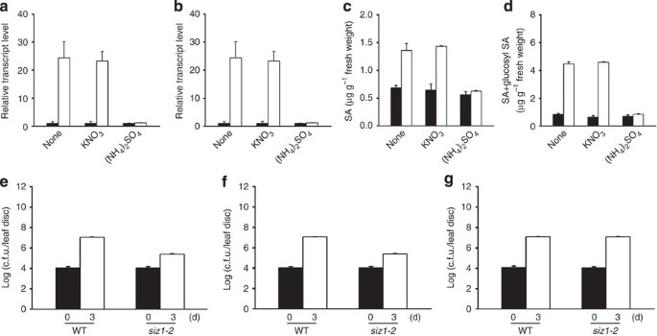Figure 8: Recovery of SA content and disease resistance to bacterial pathogens ofsiz1-2plants to WT levels by exogenous ammonium. The effect of nitrate or ammonium on transcript levels of the pathogenesis-related genesPR1andPR2was examined. Total RNAs were isolated from the leaves of WT andsiz1-2plants grown for 15 days with 5 mM KNO3or (NH4)2SO4. The transcript levels ofPR1(a) andPR2(b) were examined by real-time RT–PCR. Their transcript levels in thesiz1-2plants recovered to WT levels with (NH4)2SO4treatment. Black and white bars indicate WT andsiz1-2, respectively. Levels of free and glucosyl SA were evaluated in the leaves of 15-day-old WT andsiz1-2plants grown with 5 mM KNO3or (NH4)2SO4in soil. Samples were collected, and then SA and glucosyl SA were extracted using a methanol-based method. Free SA (c) or total SA (d) content combined with free SA and glucosyl SA were analysed with high-performance liquid chromatography. SA levels in thesiz1-2plants recovered to WT levels with (NH4)2SO4treatment. Results are expressed as means±s.d. (n=3). Black and white bars indicate WT andsiz1-2, respectively. (e–g) Effect of nitrate or ammonium on bacterial pathogen infection insiz1-2plants was also investigated. Fifteen-day-old WT andsiz1-2plants grown in soil treated with 5 mM KNO3or (NH4)2SO4were infected withP. syringaeDG3 at OD600=0.0001. The samples were collected after 3 days. The bacterial concentration was examined in leaves of WT andsiz1-2plants. (e) Non-treated WT andsiz1-2mutants. (f) KNO3-treated WT andsiz1-2mutants. (g) (NH4)2SO4-treated WT andsiz1-2mutants. The amount in (NH4)2SO4-treatedsiz1-2plants recovered to WT amounts. Values of colony-forming units (c.f.u.) represent mean±s.d. (n=8). Figure 8: Recovery of SA content and disease resistance to bacterial pathogens of siz1-2 plants to WT levels by exogenous ammonium. The effect of nitrate or ammonium on transcript levels of the pathogenesis-related genes PR1 and PR2 was examined. Total RNAs were isolated from the leaves of WT and siz1-2 plants grown for 15 days with 5 mM KNO 3 or (NH 4 ) 2 SO 4 . The transcript levels of PR1 ( a ) and PR2 ( b ) were examined by real-time RT–PCR. Their transcript levels in the siz1-2 plants recovered to WT levels with (NH 4 ) 2 SO 4 treatment. Black and white bars indicate WT and siz1-2 , respectively. Levels of free and glucosyl SA were evaluated in the leaves of 15-day-old WT and siz1-2 plants grown with 5 mM KNO 3 or (NH 4 ) 2 SO 4 in soil. Samples were collected, and then SA and glucosyl SA were extracted using a methanol-based method. Free SA ( c ) or total SA ( d ) content combined with free SA and glucosyl SA were analysed with high-performance liquid chromatography. SA levels in the siz1-2 plants recovered to WT levels with (NH 4 ) 2 SO 4 treatment. Results are expressed as means±s.d. ( n =3). Black and white bars indicate WT and siz1-2 , respectively. ( e – g ) Effect of nitrate or ammonium on bacterial pathogen infection in siz1-2 plants was also investigated. Fifteen-day-old WT and siz1-2 plants grown in soil treated with 5 mM KNO 3 or (NH 4 ) 2 SO 4 were infected with P. syringae DG3 at OD 600 =0.0001. The samples were collected after 3 days. The bacterial concentration was examined in leaves of WT and siz1-2 plants. ( e ) Non-treated WT and siz1-2 mutants. ( f ) KNO 3 -treated WT and siz1-2 mutants. ( g ) (NH 4 ) 2 SO 4 -treated WT and siz1-2 mutants. The amount in (NH 4 ) 2 SO 4 -treated siz1-2 plants recovered to WT amounts. Values of colony-forming units (c.f.u.) represent mean±s.d. ( n =8). Full size image In addition, the disease resistance against a bacterial pathogen in siz1-2 plants grown in soil containing an ammonium source was evaluated. The results showed that the susceptibility to Pseudomonas syringae DG3 was restored in ammonium-supplied siz1-2 plants ( Fig. 8e–g ). In this study, we demonstrate that nitrogen assimilation through nitrate reduction in Arabidopsis is modulated by AtSIZ1. AtSIZ1 is expressed in almost all plant tissues [16] , where it regulates cell expansion and proliferation [16] , [21] and responds to nutrient deficiency, various stresses and several developmental processes [14] , [15] , [16] , [17] , [19] , [20] , [21] . In addition, massive identification studies of SUMO conjugates in Arabidopsis have suggested that AtSIZ1 must be a central coordinator of numerous events, including basic gene expression and metabolism [25] , [26] . Nitrogen, potassium and phosphate are absolutely required for plant growth as essential nutrients. Therefore, the effect of these fertilizers on the growth of the mutant plants was examined because of the severe dwarfism of siz1-2 plants. The phenotypes were recovered to WT phenotypes with only exogenous ammonium, but not with nitrate ( Fig. 1 ; Supplementary Fig. S1 ), which suggests that the dwarf phenotypes of the siz1-2 plants may be caused by incomplete nitrate reduction due to the decreased activity or stability of NR. The results showed that the nitrogen content and NR activity were low in siz1-2 plants, while the nitrate level was high ( Fig. 2a–f ). This finding led us to analyse the functional regulation of NIA1 and NIA2 by AtSIZ1. Pull-down and yeast two-hybrid assays showed strong interactions between AtSIZ1 and NIA1 or NIA2 ( Supplementary Fig. S5a,b ). The in vitro sumoylation reaction ( Fig. 3a,b ) and in vivo bacterial infiltration assays of Arabidopsis ( Fig. 3c,d ) demonstrated that both NIA1 and NIA2 are sumoylated and their sumoylation depends on the E3 SUMO ligase AtSIZ1. These findings strongly suggest that the NR activity of both proteins must be regulated by sumoylation through the SUMO ligase activity of AtSIZ1. Studies in some eukaryotes have shown that SUMO conjugation can directly regulate the activities of target proteins, such as the binding of receptors to substrates or transcription factors to promoters. For example, the sumoylation of androgen receptor reduces its hormone-induced transcriptional activity [37] . Sumoylation of peroxisome proliferator-activated receptor g-coactivator-1α attenuates its function [38] . Sumoylation of the heat-shock factors HSF1 and HSF2 (refs 39 , 40 ) stimulates their DNA-binding activity. By contrast, sumoylation downregulates the transcriptional activation potency of some transcription factors, such as Sp3 and c-Myb [41] , [42] . Interestingly, a few studies have shown that sumoylation alters enzyme catalytic activity in animals. The sumoylation of DNMT1 and PTP1B enhances DNA methyltransferase activity and reduces phosphatase activity, respectively [43] , [44] . The sumoylation of Iκ-Bα (nuclear factor of kappa light polypeptide gene enhancer in B cells inhibitor, alpha) protects Iκ-Bα from degradation [45] , which indicates that SUMO modification can stabilize target proteins. However, no study has shown that SUMO conjugation to target proteins modulates the activity of enzymes that catalyse the conversion of substrates to products in plants. Sumoylation has been reported for several proteins in plants, including AtMYB30, PHR1, ICE1, GTE3, FLD, TPL, AtSIZ1 and AtSCE1 (refs 14 , 15 , 20 , 21 , 25 , 26 , 46 , 47 ). The sumoylations of FLD and TPL have been confirmed in vivo , although their E3 SUMO ligases have not been identified. The sumoylations of PHR1, ICE1 and GTE3 by AtSIZ1 were confirmed only in vitro . The sumoylations of the other mentioned proteins have been confirmed only in an E. coli system without E3 SUMO ligase. Recently, Peng et al . [48] reported that nitrogen limitation adaptation, a RING-type ubiquitin ligase, functions as a positive regulator that controls the adaptation of Arabidopsis to nitrogen limitations. However, the targets for nitrogen limitation adaptation or other factors involved in potential posttranslational control remain unclear. Our data showed that sumoylated NIA1 and NIA2 can form homodimers ( Supplementary Fig. S10 ), and the sumoylation of NIA1 and NIA2 by AtSIZ1 dramatically increases their nitrite production activities ( Fig. 4b–e ). These findings provide the first direct evidence of the effect of sumoylation on catalytic activity in plants. It has been shown that siz1-2 plants flower early [21] . The NR double mutant nia1/nia2 also displays an early flowering phenotype, due to its reduced NO content during vegetative growth [8] , [33] . Notably, our data showed that the siz1-2 plants contain low amounts of NO ( Fig. 2g,h ), which supports previous reports of early flowering [21] . Thus, we can cautiously conclude that the early flowering phenotype of siz1-2 plants comes from the low amount of NO, which is the result of decreased NR activity due to a lack of sumoylation. The SUMO protease mutant esd4 was shown previously to flower early in short days [13] . A double mutant missing SUMO1 and SUMO2 is not viable, and T-DNA insertion mutants affecting the single genes encoding the E1 subunit SAE2 and the E2 SCE1 are embryonic lethal [49] . The siz1-2 plants show abnormal seed development, shorter silique length, fewer seeds and growth arrest. These phenotypes of siz1-2 plants were recovered to WT phenotypes with the application of exogenous ammonium ( Supplementary Fig. S2 and Table S1 ), which indicates that nitrate reduction is an important mechanism for reproductive organ development. NR inactivation is mediated by phosphorylation [50] . Mutation analysis of the phosphorylation site of tobacco NR results in constitutive activation of the enzyme, high nitrite excretion and NO emission [51] , [52] . Together, these results indicate that phosphorylation also has an important role in reversibly modulating NR activity. It has also been suggested that NR can regulate secondary metabolism, hormone metabolism and transport, protein synthesis, signal-transduction pathways, pathways for the production of reducing equivalents and nitrate assimilation [53] . Thus, it may be that NR activity can be controlled by sumoylation or phosphorylation to exert its function effectively in various plant developmental processes. In conclusion, our work shows that sumoylation by AtSIZ1 stimulates NIA1 and NIA2 activities, and that the growth defects of siz1-2 are caused by low NR activity-induced limitations in the supply of ammonia owing to a defect in SUMO conjugation. Sumoylation, together with phosphorylation, is therefore a critical protein modification for the regulation of Arabidopsis NR activity, and sumoylation of target proteins by AtSIZ1 has an essential role in plant development through its effect on nitrogen assimilation. Plant material and culture conditions The Arabidopsis thaliana Columbia-0 (Col0) ecotype (WT) and the T-DNA insertion mutant plants siz1-2 , nia1 , nia2 and nia1/nia2 were used. Plants were grown in fully automated growth chambers under 16 h illumination either on 0.75% agar media containing Murashige and Skoog (MS) salts, 0.5 g l −1 Mes and 10 g l −1 sucrose, or on soil. Plants were maintained at 22 °C during the light period and at 20 °C during the dark period. To investigate the effect of different nitrogen sources, WT and mutant seeds were germinated and grown on MS agar media. After 4 days, seedlings were transferred into soil. A solution containing K 2 SO 4 , KNO 3 , KCl, NaNO 3 , NaCl, NaH 2 PO 4 , (NH 4 ) 2 SO 4 and NH 4 NO 3 (5 mM each) was added at 10-day intervals. To assess the effect of nitrogen on root growth, different nitrogen sources were added to the MS media. To examine chlorate sensitivity, WT and siz1-2 seeds were germinated on MS media. After 4 days, seedlings were transferred into soil and treated with 0.01 or 0.05 mM KClO 3 at 10-day intervals. All of the experiments, including enzymatic assays, were repeated three times (or more than three times, where indicated) if not mentioned further. Sumoylation assays In vitro sumoylation was performed in 30 μl of reaction buffer (200 mM HEPES (pH 7.5), 5 mM MgCl 2 , 2 mM ATP) with 500 ng of GST-SIZ1, 50 ng of His 6 -AtSAE1b, 50 ng of His 6 -AtSAE2, 50 ng of His 6 -AtSCE1, 8 μg of His 6 -AtSUMO1-GG and 100 ng of GST-NIA1 (or NIA2)-Myc and/or 100 ng of GST-mNIA1 (or mNIA2)-Myc. After incubation for 3 h at 30 °C, the reaction mixtures were separated on an 8% SDS–polyacrylamide gel. Sumoylated GST-NIA1-Myc and GST-NIA2-Myc were detected by immunoblot analysis using an anti-Myc antibody (0.2 μg ml −1 , Santa Cruz Biotechnology). For in vivo sumoylation assays, different combinations of Agrobacterium transformed with 35S-Myc-AtSIZ1 , 35S-FLAG-NIA1 (or mNIA1 ), 35S-FLAG-NIA2 (or mNIA2 ) and 35S-HA 3 -AtSUMO1 were infiltrated into N. benthamiana or WT Arabidopsis and siz1-2 plants. After 3 days, the total proteins were extracted from each sample and immunoprecipitated with an anti-haemagglutinin antibody (1 μg ml −1 , Santa Cruz Biotechnology) in a buffer containing 50 mM Tris–HCl (pH 8.0), 150 mM NaCl, 10% glycerol, 1% NP-40, 2 mM EDTA, 1 mM phenylmethyl sulphonyl fluoride (PMSF), and a protease inhibitor cocktail (Promega). Sumoylated NIA1 and NIA2 were detected by immunoblotting with an anti-FLAG antibody (0.5 μg ml −1 , Sigma-Aldrich) after IP. Effect of sumoylation on dimerization of NR To investigate whether non-sumoylated NIA1 or NIA2 can form dimers, different combinations of Agrobacterium transformed with 35S-FLAG-NIA1 (or mNIA1 ), 35S-FLAG-NIA2 (or mNIA2 ), 35S-Myc-NIA1 (or mNIA1 ), 35S-Myc-NIA2 (or mNIA2 ) and 35S-HA 3 -AtSUMO1 were infiltrated into N. benthamiana . After 3 days, total protein was extracted with a buffer containing 50 mM Tris–HCl (pH 8.0), 100 mM NaCl, 1 mM dithiothreitol, 1% Triton X-100 and protease inhibitor cocktail (Promega). Each protein extract containing Myc- and FLAG-tagged NIA1 or Myc- and FLAG-tagged NIA2 was mixed, immunoprecipitated with anti-Myc (1 μg ml −1 ) or anti-FLAG (2.5 μg ml −1 ) antibodies, and the protein interactions were examined by immunoblotting with anti-Myc (0.2 μg ml −1 ) or anti-FLAG (0.5 μg ml −1 ) antibodies. The mixtures were also immunoprecipitated with an anti-haemagglutinin antibody, (1 μg ml −1 ) and the sumoylation of NIA1 or NIA2 was examined by immunoblotting with anti-Myc (0.2 μg ml −1 ) or anti-FLAG (0.5 μg ml −1 ) antibodies. To investigate whether sumoylated NIA1 or NIA2 can form dimers, different combinations of the Agrobacterium transformed with XVE-His 6 -HA 3 -AtSUMO1/35S-FLAG-NIA1 (or mNIA1 ) or XVE-His 6 -HA 3 -AtSUMO1/35S-Myc-NIA1 (or mNIA1 ), and XVE-His 6 -HA 3 -AtSUMO1/35S-FLAG-NIA2 (or mNIA2 ) or XVE-His 6 -HA 3 -AtSUMO1/35S-Myc-NIA2 (or mNIA2 ) and 10 μM of β-estradiol were infiltrated into N. benthamiana . After overnight incubation, the leaves were injected again with 10 μM of β-estradiol and further incubated for 3 d. The infiltrated leaves were collected and total protein was extracted with the buffer described above. After the sumoylated NIA1 and NIA2 were detected by immunoblotting with anti-Myc (0.2 μg ml −1 ) or anti-FLAG (0.5 μg ml −1 ) antibodies using the fraction purified with a Ni 2+ -NTA resin, the fractions were mixed and immunoprecipitated with anti-Myc (1 μg ml −1 ) or anti-FLAG (2.5 μg ml −1 ) antibodies. Finally, sumoylated NIA1 or NIA2 was detected by western blotting with anti-Myc (0.2 μg ml −1 ) or anti-FLAG (0.5 μg ml −1 ) antibodies. NR assay The NR activity of plant crude extracts was assayed using leaves of WT or siz1-2 plants. Briefly, leaves of WT or siz1-2 plants were homogenized in extraction buffer (250 mM Tris–HCl (pH 8.0), 1 mM EDTA, 1 μM Na 2 MoO 4 , 5 μM flavin adenine dinucleotide, 3 mM dithiothreitol, 1% BSA, 12 mM β-mercaptoethanol and 250 μM PMSF). After centrifugation at 13,000 r.p.m. for 5 min, supernatants were collected and added to reaction buffer (40 mM NaNO 3 , 80 mM Na 2 HPO 4 , 20 mM NaH 2 PO 4 (pH 7.5) and 0.2 mM NADH). The reaction was stopped by the addition of 1% sulphanilamide and 0.05% N -(1-napthyl) ethylenediamine hydrochloride after further incubation for 2 h at room temperature. The concentration of nitrite was determined by measuring the absorbance of the reaction mixture at 540 nm [56] . Measurement of the specific activity of NR Combinations of Agrobacterium transformed with NIA and SUMO constructs ( 35S-His 10 -NIA1 ( mNIA1 ) -FLAG 3 , 35S-His 10 -NIA2 (or mNIA2 ) -FLAG 3 and 35S-HA 3 -AtSUMO1 ) were infiltrated into WT and siz1-2 plants. After 3 days, samples were collected and total proteins were extracted with a buffer containing 50 mM Tris–HCl (pH 8.0), 150 mM NaCl, 10% glycerol, 1% NP-40, 2 mM EDTA, 1 mM PMSF and a proteinase inhibitor cocktail. Sumoylated or non-sumoylated NIA1 and NIA2 proteins were purified on Ni 2+ -NTA resins (Qiagen) in accordance with the manufacturer's instructions. For activity assays, 50 ng of purified protein were added to a reaction buffer containing 40 mM NaNO 3 , 80 mM Na 2 HPO 4 , 20 mM NaH 2 PO 4 (pH 7.5) and 0.2 mM NADH. After incubation for 2 h at room temperature, the reaction was stopped by the addition of 1% sulphanilamide and 0.05% N -(1-napthyl) ethylenediamine hydrochloride. The specific activity was calculated from the concentration of nitrite determined through the measurement of the absorbance of the reaction mixture at 540 nm [54] . Measurement of in situ NO The root tip and centre (about 0.5 cm from the root tip) were excised from the roots of WT or siz1-2 plants grown in MS containing 5 mM KNO 3 for 15 days. After treatment with 5 μM DAF-FM DA (3-amino, 4-aminomethyl-2′,7′-difluorescein, diacetate, a fluorescent NO indicator dye) for 15 min, samples were washed with HEPES buffer (pH 7.4) for 10 min. Fluorescence was observed with a fluorescence microscope (excitation 495 nm, emission 515 nm; Carl Zeiss-LSM510). Examination of NR level and stability Total proteins were extracted from the leaves of WT, siz1-2 , nia1 , nia2 and nia1/nia2 plants grown for 10 days in MS media. After 8% SDS–PAGE, the levels of the NRs NIA1 and NIA2 were examined by immunoblotting with a cucumber anti-NR antibody (antibodies-Online). To estimate the effect of AtSIZ1 on NR stability, WT and siz1-2 plants grown on MS media for 15 days were treated with 100 μM cycloheximide for 1 h. Total RNAs were isolated, and the transcript levels of NIA1 and NIA2 were examined by real-time RT–PCR. To evaluate the NR level, WT and siz1-2 plants grown on MS media for 15 days were treated with 100 μM cycloheximide for 8 h, and the samples were collected at the indicated time points. The total proteins were extracted, and the NRs were detected by immunoblotting with the cucumber anti-NR antibody (0.5 μg ml −1 ). Pathogen inoculation For pathogen inoculation, WT and siz1-2 plants grown for 15 days in soil treated with K 2 SO 4 , KNO 3 and (NH 4 ) 2 SO 4 (5 mM each) were infected with the bacterial pathogen P. syringae DG3 (ref. 55 ) as follows. The bacteria were grown at 28°C in King's liquid medium containing 50 μg ml −1 rifampicin and kanamycin. After absorbance at 600 nm reached 1.0, the bacteria were centrifuged, resuspended in 10 mM MgCl 2 (OD 600 =0.0001), and hand-inoculated into leaves with 1-ml blunt syringes. The plants were covered with a plastic dome for 3 days to subject them to conditions of humidity. Eight leaves from four WT or siz1-2 plants were collected, punched, and ground in 10 mM MgCl 2 . After serial dilutions with 10 mM MgCl 2 , the bacterial solutions were plated onto King's medium containing the appropriate antibiotics. After incubation for 3 days, colonies were counted. Determination of SA and its conjugates Salicylic acid and the SA-conjugate glucosyl SA were extracted from leaves of 15-day-old WT and siz1-2 plants grown in soil treated with K 2 SO 4 , KNO 3 and (NH 4 ) 2 SO 4 (5 mM each). The leaves were ground to a fine powder, and SA was extracted sequentially with 90 and 100% methanol. After centrifugation, the methanol-containing supernatants were vacuum-dried and resuspended in 5% trichloroacetic acid. After partition with two volumes of ethyl acetate/cyclopentane/isopropanol (100:99:1, vol/vol) and drying under nitrogen gas, the pellets were resuspended in 70% methanol. Finally, the SA content was determined by high-performance liquid chromatography [56] . For free SA and glucosyl SA extraction, vacuum-dried samples were resuspended in 5 mM sodium acetate buffer (pH 5.5) containing 80 units g −1 fresh weight β-glucosidase (Sigma). After incubation for 90 min at 37 °C, the reaction was stopped with the addition of 5% trichloroacetic acid. After partition, drying and resuspension, the amounts of free and glucosyl SA were determined by high-performance liquid chromatography. Experimental procedures about construction and purification of recombinant plasmids and proteins, yeast two-hybrid, in vitro binding assay, measurement of nitrogen and nitrate contents, real-time RT–PCR and chlorate resistance are described in the Supplementary Methods . How to cite this article: Park, B.S. et al . Arabidopsis nitrate reductase activity is stimulated by the E3 SUMO ligase AtSIZ1. Nat. Commun. 2:400 doi: 10.1038/natcomms1408 (2011).